Observation of long-lived interlayer excitons in monolayer MoSe2–WSe2heterostructures Van der Waals bound heterostructures constructed with two-dimensional materials, such as graphene, boron nitride and transition metal dichalcogenides, have sparked wide interest in device physics and technologies at the two-dimensional limit. One highly coveted heterostructure is that of differing monolayer transition metal dichalcogenides with type-II band alignment, with bound electrons and holes localized in individual monolayers, that is, interlayer excitons. Here, we report the observation of interlayer excitons in monolayer MoSe 2 –WSe 2 heterostructures by photoluminescence and photoluminescence excitation spectroscopy. We find that their energy and luminescence intensity are highly tunable by an applied vertical gate voltage. Moreover, we measure an interlayer exciton lifetime of ~1.8 ns, an order of magnitude longer than intralayer excitons in monolayers. Our work demonstrates optical pumping of interlayer electric polarization, which may provoke further exploration of interlayer exciton condensation, as well as new applications in two-dimensional lasers, light-emitting diodes and photovoltaic devices. The recently developed ability to vertically assemble different two-dimensional (2D) materials heralds a new realm of device physics based on van der Waals heterostructures (HSs) [1] . The most successful example to date is the vertical integration of graphene on boron nitride. Such novel HSs not only markedly enhance graphene’s electronic properties [2] , but also give rise to superlattice structures demonstrating exotic physical phenomena [3] , [4] , [5] . A fascinating counterpart to gapless graphene is a class of monolayer direct bandgap semiconductors, namely transition metal dichalcogenides (TMDs) [6] , [7] , [8] . Due to the large binding energy in these 2D semiconductors, excitons dominate the optical response, exhibiting strong light–matter interactions that are electrically tunable [9] , [10] . The discovery of excitonic valley physics [11] , [12] , [13] , [14] , [15] and strongly coupled spin and pseudospin physics [16] , [17] in 2D TMDs opens up new possibilities for device concepts not possible in other material systems. Monolayer TMDs have the chemical formula MX 2 where the M is tungsten (W) or molybdenum (Mo), and the X is sulfur (S) or selenium (Se). Although these TMDs share the same crystalline structure, their physical properties, such as bandgap, exciton resonance and spin–orbit coupling strength, can vary significantly. Therefore, an intriguing possibility is to stack different TMD monolayers on top of one another to form 2D HSs . First-principle calculations show that heterojunctions formed between monolayer tungsten and molybdenum dichalcogenides have type-II band alignment [18] , [19] , [20] . Recently, this has been confirmed by X-ray photoelectron spectroscopy and scanning tunnelling spectroscopy [21] . Since the Coulomb binding energy in 2D TMDs is much stronger than in conventional semiconductors, it is possible to realize interlayer excitonic states in van der Waals bound heterobilayers, that is, bound electrons and holes that are localized in different layers. Such interlayer excitons have been intensely pursued in bilayer graphene for possible exciton condensation [22] , but direct optical observation demonstrating the existence of such excitons is challenging owing to the lack of a sizable bandgap in graphene. Monolayer TMDs with bandgaps in the visible range provide the opportunity to optically pump interlayer excitons, which can be directly observed through photoluminescence (PL) measurements. In this report, we present direct observation of interlayer excitons in vertically stacked monolayer MoSe 2 –WSe 2 HSs. We show that interlayer exciton PL is enhanced under optical excitation resonant with the intralayer excitons in isolated monolayers, consistent with the interlayer charge transfer resulting from the underlying type-II band structure. We demonstrate the tuning of the interlayer exciton energy by applying a vertical gate voltage, which is consistent with the permanent out-of-plane electric dipole nature of interlayer excitons. Moreover, we find a blue shift in PL energy at increasing excitation power, a hallmark of repulsive dipole–dipole interactions between spatially indirect excitons. Finally, time-resolved PL measurements yield a lifetime of 1.8 ns, which is at least an order of magnitude longer than that of intralayer excitons. Our work shows that monolayer semiconducting HSs are a promising platform for exploring new optoelectronic phenomena. MoSe 2 –WSe 2 HS photoluminescence HSs are prepared by standard polymethyl methacrylate (PMMA) transfer techniques using mechanically exfoliated monolayers of WSe 2 and MoSe 2 (see Methods). Since there is no effort made to match the crystal lattices of the two monolayers, the obtained HSs are considered incommensurate. An idealized depiction of the vertical MoSe 2 –WSe 2 HS is shown in Fig. 1a . We have fabricated six devices that all show similar results as those reported below. The data presented here are from two independent MoSe 2 –WSe 2 HSs, labelled device 1 and device 2. 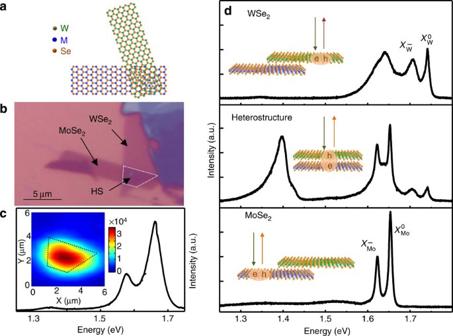Figure 1: Intralayer and interlayer excitons of a monolayer MoSe2–WSe2vertical heterostructure. (a) Cartoon depiction of a MoSe2–WSe2heterostructure (HS). (b) Microscope image of a MoSe2–WSe2HS (device 1) with a white dashed line outlining the HS region. (c) Room-temperature photoluminescence of the heterostructure under 20 μW laser excitation at 2.33 eV. Inset: spatial map of integrated PL intensity from the low-energy peak (1.273–1.400 eV), which is only appreciable in the heterostructure area, outlined by the dashed black line. (d) Photoluminescence of individual monolayers and the HS at 20 K under 20 μW excitation at 1.88 eV (plotted on the same scale). Figure 1b shows an optical micrograph of device 1, which has individual monolayers, as well as a large area of vertically stacked HS. This device architecture allows for the comparison of the excitonic spectrum of individual monolayers with that of the HS region, allowing for a controlled identification of spectral changes resulting from interlayer coupling. Figure 1: Intralayer and interlayer excitons of a monolayer MoSe 2 –WSe 2 vertical heterostructure. ( a ) Cartoon depiction of a MoSe 2 –WSe 2 heterostructure (HS). ( b ) Microscope image of a MoSe 2 –WSe 2 HS (device 1) with a white dashed line outlining the HS region. ( c ) Room-temperature photoluminescence of the heterostructure under 20 μW laser excitation at 2.33 eV. Inset: spatial map of integrated PL intensity from the low-energy peak (1.273–1.400 eV), which is only appreciable in the heterostructure area, outlined by the dashed black line. ( d ) Photoluminescence of individual monolayers and the HS at 20 K under 20 μW excitation at 1.88 eV (plotted on the same scale). Full size image We characterize the MoSe 2 –WSe 2 monolayers and HS using PL measurements. Inspection of the PL from the HS at room temperature reveals three dominant spectral features ( Fig. 1c ). The emission at 1.65 and 1.57 eV corresponds to the excitonic states from monolayer WSe 2 and MoSe 2 (refs 10 , 15 ), respectively. PL from the HS region, outlined by the dashed white line in Fig. 1a , reveals a distinct spectral feature at 1.35 eV ( X I ). Two-dimensional mapping of the spectrally integrated PL from X I shows that it is isolated entirely to the HS region (inset, Fig. 1c ), with highly uniform peak intensity and spectral position ( Supplementary Materials 1 ). Low-temperature characterization of the HS is performed with 1.88 eV laser excitation at 20 K. PL from individual monolayer WSe 2 (top), MoSe 2 (bottom) and the HS area (middle) are shown with the same scale in Fig. 1d . At low temperature, the intralayer neutral ( X M o ) and charged ( X M − ) excitons are resolved [10] , [15] , where M labels either W or Mo. Comparison of the three spectra shows that both intralayer X M o and X M − exist in the HS with emission at the same energy as from isolated monolayers, demonstrating the preservation of intralayer excitons in the HS region. PL from X I becomes more pronounced and is comparable to the intralayer excitons at low temperature. We note that the X I energy position has variation across the pool of HS samples we have studied ( Supplementary Fig. 1 ), which we attribute to differences in the interlayer separation, possibly due to imperfect transfer and a different twisting angle between monolayers. We further perform PL excitation (PLE) spectroscopy to investigate the correlation between X I and intralayer excitons. A narrow bandwidth (<50 kHz) frequency tunable laser is swept across the energy resonances of intralayer excitons (from 1.6 to 1.75 eV) while monitoring X I PL response. 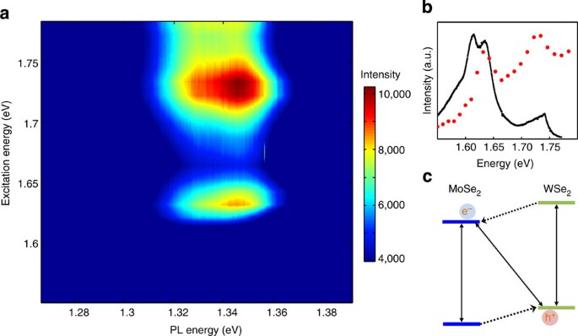Figure 2: Photoluminescence excitation spectroscopy of the interlayer exciton at 20 K. (a) PLE intensity plot of the heterostructure region with an excitation power of 30 μW and 5 s charge-coupled device CCD integration time. (b) Spectrally integrated PLE response (red dots) overlaid on PL (black line) with 100 μW excitation at 1.88 eV. (c) Type-II semiconductor band alignment diagram for the 2D MoSe2–WSe2heterojunction. Figure 2a shows an intensity plot of X I emission as a function of photoexcitation energy from device 2. We clearly observe the enhancement of X I emission when the excitation energy is resonant with intralayer exciton states ( Fig. 2b ). Figure 2: Photoluminescence excitation spectroscopy of the interlayer exciton at 20 K. ( a ) PLE intensity plot of the heterostructure region with an excitation power of 30 μW and 5 s charge-coupled device CCD integration time. ( b ) Spectrally integrated PLE response (red dots) overlaid on PL (black line) with 100 μW excitation at 1.88 eV. ( c ) Type-II semiconductor band alignment diagram for the 2D MoSe 2 –WSe 2 heterojunction. Full size image Now we discuss the origin of X I . Since X I has never been observed in our exfoliated monolayer and bilayer samples, if its origin were related to defects, they must be introduced by the fabrication process. This would result in sample-dependent X I properties with non-uniform spatial dependence. However, our data show that key physical properties of X I , such as the resonance energy and intensity, are spatially uniform and isolated to the HS region (inset of Fig. 1c and Supplementary Fig. 2 ). In addition, X I has not been observed in WSe 2 –WSe 2 homostructures constructed from exfoliated or physical vapor deposition (PVD) grown monolayers ( Supplementary Fig. 3 ). All these facts suggest that X I is not a defect-related exciton. Instead, the experimental results support the observation of an interlayer exciton. Due to the type-II band alignment of the MoSe 2 –WSe 2 HS [18] , [19] , [20] , as shown in Fig. 2c , photoexcited electrons and holes will relax (dashed lines) to the conduction band edge of MoSe 2 and the valence band edge of WSe 2 , respectively. The Coulomb attraction between electrons in the MoSe 2 and holes in the WSe 2 gives rise to an interlayer exciton, X I , analogous to spatially indirect excitons in coupled quantum wells. The interlayer coupling yields the lowest energy bright exciton in the HS, which is consistent with the temperature dependence of X I PL, that is, it increases as temperature decreases ( Supplementary Fig. 4 ). From the intralayer and interlayer exciton spectral positions, we can infer the band offsets between the WSe 2 and MoSe 2 monolayers ( Fig. 2c ). The energy difference between X W and X I at room temperature is 310 meV. Considering the smaller binding energy of interlayer than intralayer excitons, this sets a lower bound on the conduction band offset. The energy difference between X M and X I then provides a lower bound on the valence band offset of 230 meV. This value is consistent with the valence band offset of 228 meV found in MoS 2 –WSe 2 HSs by micro X-ray photoelectron spectroscopy and scanning tunnelling spectroscopy measurements [21] . This experimental evidence strongly corroborates X I as an interlayer exciton. The observation of bright interlayer excitons in monolayer semiconducting HSs is of central importance, and the remainder of this paper will focus on their physical properties resulting from their spatially indirect nature and the underlying type-II band alignment. Electrical control of the interlayer exciton Applying a vertical gate bias across the HS demonstrates that the emission energy of the interlayer exciton is highly electrically tunable. 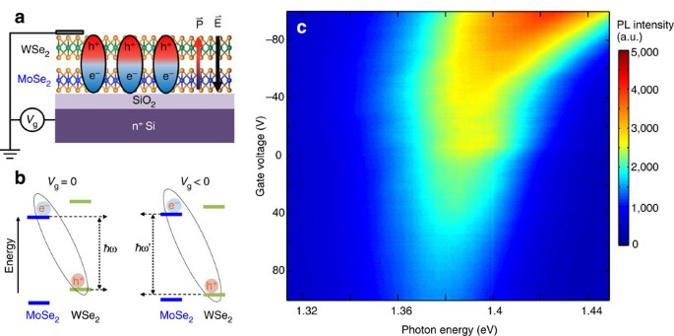Figure 3: Gate control of the interlayer exciton and band alignment. (a) Device 2 geometry. The interlayer exciton has a permanent dipole, corresponding to an out-of-plane electric polarization. (b) Electrostatic control of the band alignment and the interlayer exciton resonance. (c) Colourmap of interlayer exciton photoluminescence as a function of applied gate voltage under 70 μW excitation at 1.744 eV, 1 s integration time. Figure 3a shows the contact geometry of device 2, where an indium contact has been fabricated on the WSe 2 layer, which is vertically stacked on top of the MoSe 2 . The HS is on SiO 2 , which provides insulation from the heavily doped silicon backgate. Electrostatic doping is performed on the HS by grounding the indium contact and applying a voltage to the backgate ( V g ). Figure 3c shows the interlayer exciton PL intensity as V g is varied from +100 to −100 V. Over this range, the peak centre blue shifts by about 45 meV. Subsequent measurements on an inverted analogue of device 2, where the stacking order of MoSe 2 and WSe 2 is reversed, shows the peak centre red shift by about 60 meV as V g is varied from +70 to −70 V ( Supplementary Fig. 5 ). Figure 3: Gate control of the interlayer exciton and band alignment. ( a ) Device 2 geometry. The interlayer exciton has a permanent dipole, corresponding to an out-of-plane electric polarization. ( b ) Electrostatic control of the band alignment and the interlayer exciton resonance. ( c ) Colourmap of interlayer exciton photoluminescence as a function of applied gate voltage under 70 μW excitation at 1.744 eV, 1 s integration time. Full size image The gate dependence of X I is consistent with that expected for the interlayer exciton, which maintains a dipole pointing from MoSe 2 to WSe 2 ( Fig. 3a ). At negative V g , the electric field reduces the relative band-offset between the MoSe 2 and WSe 2 in device 2, increasing the energy separation between the MoSe 2 conduction band and the WSe 2 valence band, as shown in Fig. 3b,c . The interaction of the field and the anti-aligned dipole of the interlayer exciton thus results in the observed blue shift in the energy of PL from X I . Conversely, when MoSe 2 is located on top of WSe 2 , the field effect increases the relative band-offset at negative V g , manifesting the observed red shift in X I PL ( Supplementary Fig. 5 ). The electrical control of the energy of X I confirms the direction of its permanent dipole. On the basis of this electrical field and dipole interaction picture, we would expect that the X I PL intensity in devices 2 and 3 should have opposite behaviours. However, we observe that the X I PL increases as gate voltage decreases in both devices. This observation shows that in addition to the electrical field effect, carrier doping may play a significant role in tuning X I intensity. We expect devices with both top and bottom gates may further elucidate the observed phenomena. Power dependence and lifetime of interlayer exciton PL The interlayer exciton PLE spectrum as a function of laser power with excitation energy in resonance with X W o reveals several properties of the X I . Inspection of the normalized PLE intensity ( Fig. 4a ) shows the evolution of a doublet in the interlayer exciton spectrum, highlighted by the red and green bi-Lorentzian fits. Both peaks of the doublet display a consistent blue shift with increased laser intensity, shown by the dashed arrows in Fig. 4a , which are included as a guide to the eye. The spectrally integrated intensity of X I also exhibits a strong saturation as a function of laser power, as shown in Fig. 4b (absolute PL intensity shown in Supplementary Fig. 6 ). The sublinear power response of X I for excitation powers above 0.5 μW is distinctly different than that for the intralayer excitons in isolated monolayers, which display a saturation power threshold of about 80 μW ( Supplementary Fig. 7 ). 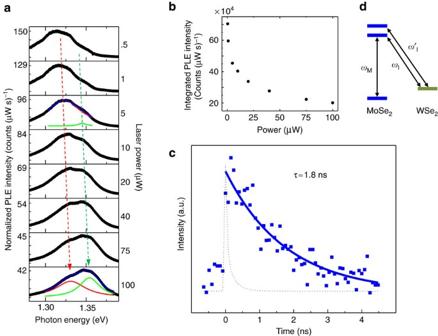Figure 4: Power-dependent photoluminescence of interlayer exciton and its lifetime at 20 K. (a) Power dependence of the interlayer exciton for 1.722 eV excitation with a bi-Lorentzian fit to the 5 and 100 μW plots, normalized for power and charge-coupled device (CCD) integration time. (b) Spectrally integrated intensity of the interlayer exciton emission as a function of excitation power shows the saturation effect. (c) Time-resolved photoluminescence of the interlayer exciton (1.35 eV) shows a lifetime of about 1.8 ns. The dashed curve is the instrument response to the excitation laser pulse. (d) Illustration of the heterojunction band diagram, including the spin levels of the MoSe2conduction band. TheXIdoublet has energy splitting equal toℏ(ω′I−ωI) ≈25 meV. Figure 4: Power-dependent photoluminescence of interlayer exciton and its lifetime at 20 K. ( a ) Power dependence of the interlayer exciton for 1.722 eV excitation with a bi-Lorentzian fit to the 5 and 100 μW plots, normalized for power and charge-coupled device (CCD) integration time. ( b ) Spectrally integrated intensity of the interlayer exciton emission as a function of excitation power shows the saturation effect. ( c ) Time-resolved photoluminescence of the interlayer exciton (1.35 eV) shows a lifetime of about 1.8 ns. The dashed curve is the instrument response to the excitation laser pulse. ( d ) Illustration of the heterojunction band diagram, including the spin levels of the MoSe 2 conduction band. The X I doublet has energy splitting equal to ℏ ( ω ′ I − ω I ) ≈25 meV. Full size image The low power saturation of X I PL suggests a much longer lifetime than that of intralayer excitons. In the HS, the lifetime of the intralayer exciton is substantially reduced by the ultrafast interlayer charge hopping [23] , which is evidenced by the strong quenching of intralayer exciton PL ( Fig. 1d ; Supplementary Fig. 8 ). Moreover, the lifetime of the interlayer exciton is long, because it is the lowest energy configuration and its spatially indirect nature leads to a reduced optical dipole moment. This long lifetime is confirmed by time-resolved PL, as shown in Fig. 4c . A fit to a single exponential decay yields an interlayer exciton lifetime of 1.8±0.3 ns. This timescale is much longer than the intralayer exciton lifetime, which is on the order of tens of ps [24] , [25] , [26] , [27] . By modelling the saturation behaviour using a simplified three-level diagram, the calculated saturation intensity for the interlayer exciton is about 180 times smaller than intralayer ( Supplementary Fig. 7 ; Supplementary Discussion ), consistent with our observation of low saturation intensity of X I . We attribute the observed doublet feature in Fig. 4a to the spin-splitting of the monolayer MoSe 2 conduction band ( Fig. 4d ). This assignment is mainly based on the fact that the extracted energy difference between the doublet is ~25 meV, which agrees well with MoSe 2 conduction band splitting predicted by first-principle calculations [28] . This explanation is also supported by the evolution of the relative strength of the two peaks with increasing excitation power, as shown in Fig. 4a (similar results in device 1 with 1.88 eV excitation shown in Supplementary Fig. 9 ). At low power, the lowest energy configuration of interlayer excitons, with the electron in the lower spin-split band of MoSe 2 , is populated first. Due to phase space filling effects, the interlayer exciton configuration with the electron in the higher energy spin-split band starts to be filled at higher laser power. Consequently, the higher energy peak of the doublet becomes more prominent at higher excitation powers. The observed blue shift of X I as the excitation power increases, indicated by the dashed arrows in Fig. 4a , is a signature of the repulsive interaction between the dipole-aligned interlayer excitons ( cf. Fig. 3a ). This is a hallmark of spatially indirect excitons in gallium arsenide (GaAs) coupled quantum wells, which have been intensely studied for exciton Bose-Einstein condensation (BEC) phenomena [29] . The observation of spatially indirect interlayer excitons in a type-II semiconducting 2D HS provides an intriguing platform to explore exciton BEC, where the observed extended lifetimes and repulsive interactions are two key ingredients towards the realization of this exotic state of matter. Moreover, the extraordinarily high binding energy for excitons in this truly 2D system may provide for degenerate exciton gases at elevated temperatures compared with other material systems [30] . The long-lived interlayer exciton may also lead to new optoelectronic applications, such as photovoltaics [31] , [32] , [33] , [34] and 2D HS nanolasers. Device fabrication Monolayers of MoSe 2 are mechanically exfoliated onto 300 nm SiO 2 on heavily doped Si wafers and monolayers of WSe 2 onto a layer of PMMA atop polyvinyl alcohol on Si. Both monolayers are identified with an optical microscope and confirmed by their PL spectra. Polyvinyl alcohol is dissolved in H 2 O and the PMMA layer is then placed on a transfer loop or thin layer of polydimethylsiloxane (PDMS). The top monolayer is then placed in contact with the bottom monolayer with the aid of an optical microscope and micromanipulators. The substrate is then heated to cause the PMMA layer to release from the transfer media. The PMMA is subsequently dissolved in acetone for ~30 min and then rinsed with isopropyl alcohol. Low-temperature PL measurements Low-temperature measurements are conducted in a temperature-controlled Janis cold finger cryostat (sample in vacuum) with a diffraction-limited excitation beam diameter of ~1 μm. PL is spectrally filtered through a 0.5-m monochromator (Andor–Shamrock) and detected on a charge-coupled device (Andor—Newton). Spatial PL mapping is performed using a Mad City Labs Nano-T555 nanopositioning system. For PLE measurements, a continuous wave Ti:sapphire laser (MSquared—SolsTiS) is used for excitation and filtered from the PL signal using an 815-nm-long pass optical filter (Semrock). Electrostatic doping is accomplished with an indium drain contact deposited onto the monolayer WSe 2 region of device 2 and using the heavily doped Si as a tunable backgate. Time-resolved PL measurements For interlayer lifetime measurements, we excite the sample with a <200-fs pulsed Ti:sapphire laser (Coherent—MIRA). Interlayer PL is spectrally filtered through a 0.5-m monochromator (Princeton—Acton 2500), and detected with a fast time-correlated single-photon counting system composed of a fast (<30 ps full width at half maximum) single-photon avalanche detector (Micro Photon Devices—PDM series) and a picosecond event timer (PicoQuant—PicoHarp 300). How to cite this article: Rivera, P. et al . Observation of long-lived interlayer excitons in monolayer MoSe 2 –WSe 2 heterostructures. Nat. Commun. 6:6242 doi: 10.1038/ncomms7242 (2015).